Multimetallic catalysed radical oxidative C(sp3)–H/C(sp)–H cross-coupling between unactivated alkanes and terminal alkynes Radical involved transformations are now considered as extremely important processes in modern organic synthetic chemistry. According to the demand by atom-economic and sustainable chemistry, direct C(sp 3 )–H functionalization through radical oxidative coupling represents an appealing strategy for C–C bond formations. However, the selectivity control of reactive radical intermediates is still a great challenge in these transformations. Here we show a selective radical oxidative C(sp 3 )–H/C(sp)–H cross-coupling of unactivated alkanes with terminal alkynes by using a combined Cu/Ni/Ag catalytic system. It provides a new way to access substituted alkynes from readily available materials. Preliminary mechanistic studies suggest that this reaction proceeds through a radical process and the C(sp 3 )–H bond cleavage is the rate-limiting step. This study may have significant implications for controlling selective C–C bond formation of reactive radical intermediates by using multimetallic catalytic systems. Substituted alkynes are fundamental structural motifs in numerous natural products, bioactive molecules and functional materials [1] , [2] , [3] . They also serve as versatile intermediates in many chemical transformations. Continuous efforts have been devoted to their synthesis throughout the history of organic chemistry. During the last decades, the transition-metal-catalysed Sonogashira coupling has been proven to be one of the most popular and efficient approach for the synthesis of substituted alkynes [4] . While early studies focused on C(sp 2 )–C(sp) coupling of terminal alkynes with vinyl/aryl electrophiles, recent attention has been paid to the C(sp 3 )–C(sp) coupling of terminal alkynes with unactivated alkyl halides. In 2003, Eckhardt and Fu [5] pioneered the cross-coupling of terminal alkynes with unactivated primary bromides and iodides by using Pd/Cu synergistic catalysis with N–heterocyclic carbene ligands. Later on, this reaction protocol was extended to unactivated secondary bromides and iodides by Altenhoff et al . [6] . In 2009, Vechorkin et al . [7] applied a combined Ni/Cu catalytic system to achieve the coupling of terminal alkynes with unactivated primary halides. Similarly, a modified Ni/Cu co-catalysed system was developed by Yi et al . [8] to deal with the coupling with secondary bromides and iodides. More recently, Chen et al . [9] developed a photo–promoted, transition-metal-free protocol to couple terminal alkynes with all types of unactivated alkyl iodides. As an alternative process for achieving the direct alkynylation of terminal alkynes, our group demonstrated a Pd-catalysed oxidative cross-coupling between terminal alkynes and alkylzinc reagents for the synthesis of substituted alkynes. Echoing the pursuit of atom-economic and sustainable chemistry, direct utilization of unactivated alkanes to replace unactivated alkyl halides and alkylzinc reagents in the synthesis of substituted alkynes has great significance in terms of both concept innovation and practical application. Direct C(sp 3 )–H functionalization is a highly attractive approach for converting alkanes into functionalized organic compounds. However, the development of direct and selective methods for alkane functionalization is still in its infancy due to the low reactivity of C(sp 3 )–H bonds [10] , [11] , [12] , [13] , [14] , [15] . With the rapid development of C–H functionalization, direct C–H alkynylation with terminal alkynes has recently emerged as one of the most attractive approaches to access substituted alkynes [16] , [17] , [18] , [19] , [20] , [21] , [22] , [23] , [24] , [25] , [26] . This transformation has been considered to be challenging because of the facile homo-coupling and polymerization of terminal alkynes under oxidative conditions. Methods for the oxidative C(sp 3 )–H alkynylation of tertiary amines [27] , [28] , [29] , [30] or benzylic ethers [31] , [32] have been developed through normal cross-dehydrogenative coupling [33] pathway ( Fig. 1a ), but direct oxidative C(sp 3 )–H alkynylation of unactivated alkanes with terminal alkynes to form substituted alkynes is still a great challenge and remains undeveloped. 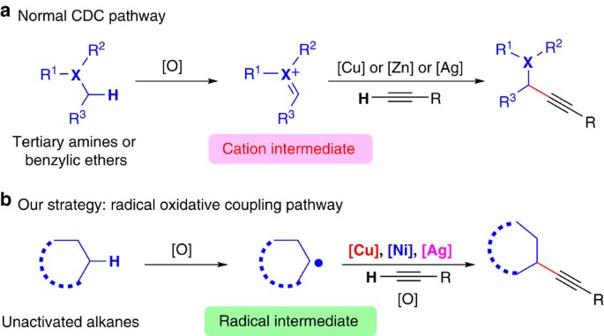Figure 1: Approaches for C(sp3)–H/C(sp)–H coupling. (a) Alkynylation of activated C(sp3)–H bonds through CDC pathway. (b) Proposed radical oxidative coupling pathway for C(sp3)–H alkynylation of unactivated alkanes with terminal alkynes. Figure 1: Approaches for C(sp 3 )–H/C(sp)–H coupling. ( a ) Alkynylation of activated C(sp 3 )–H bonds through CDC pathway. ( b ) Proposed radical oxidative coupling pathway for C(sp 3 )–H alkynylation of unactivated alkanes with terminal alkynes. Full size image Herein, we report a Cu/Ni/Ag co-catalysed oxidative C(sp 3 )–H alkynylation of unactivated alkanes with terminal alkynes. This protocol provides a new approach for the synthesis of substituted alkynes from readily available materials. Various alkanes and terminal alkynes are suitable in this transformation, affording the C(sp 3 )–C(sp) coupling product in good to high yields. Designing strategy Radicals have been widely utilized in a large range of processes such as organic synthesis, biological processes and polymerization [34] , [35] , [36] , [37] . Generally, radicals with a single electron have a strong tendency to form chemical bonds. However, selective bond formation from radical intermediates was less developed compared with the ionic intermediates. Recent achievements showed that radical cross-coupling can provide a new opportunity for the formation of C–C bonds [38] , [39] , [40] . Considering that unactivated alkanes can be converted into corresponding alkyl radicals in the presence of oxidants, we envisioned that a radical oxidative cross-coupling pathway might provide a solution for the C(sp 3 )–H/C(sp)–H cross-coupling between unactivated alkanes and terminal alkynes ( Fig. 1b ). Nevertheless, the direct coupling of an alkyl radical with terminal alkynes usually ends up with reductive addition or difunctionalization to afford internal alkenes [41] , [42] , [43] , [44] . It was difficult to control the selectivity toward direct alkynylation rather than simple addition to alkyne. To deal with this challenging transformation, we wish to report a selective radical oxidative C(sp 3 )–H/C(sp)–H cross-coupling of unactivated alkanes with terminal alkynes by using a multimetallic catalysis [45] system ( Fig. 1b ). Optimization of reaction conditions We started our research by examining the model reaction between cyclohexane ( 1a ) and p -tolylacetylene ( 2a ) under various conditions. After considerable efforts, we found that the combination of Cu(OTf) 2 , Ni(acac) 2 and AgOAc as catalysts, 1,4–bis(diphenylphosphino)butane (dppb) as ligand, and di- tert -butyl peroxide (DTBP) as oxidant in chlorobenzene at 130 °C gave the best result (see Supplementary Tables 1–5 for detailed condition optimization). A 75% GC yield could be obtained within 3 h ( Table 1 , entry 1). The effect of each reaction parameter was examined and listed in Table 1 . Both copper and nickel catalysts were crucial for this C(sp 3 )–C(sp) coupling reaction. Only 6% yield of the desired product was obtained in the absence of Ni(acac) 2 ( Table 1 , entry 2). No desired products could be observed in the absence of Cu(OTf) 2 ( Table 1 , entry 3). Instead, direct addition product 4a was obtained in 13% yield ( Fig. 2a ). Moreover, CuOTf failed to furnish the coupling product ( Table 1 , entry 4). Ligand was not indispensable for this oxidative cross-coupling reaction. A moderate yield could be obtained in the absence of ligand ( Table 1 , entry 5). Addition of bipyridine did not improve the reaction yield ( Table 1 , entry 6). PPh 3 was less effective than dppb in this transformation ( Table 1 , entry 7). Control experiments regarding the role of silver were also performed ( Table 1 , entries 8–9). In the absence of AgOAc, a good but slightly decreased yield could still be obtained ( Table 1 , entry 8). When CsOAc was used instead of AgOAc, the reaction resulted in a poor yield ( Table 1 , entry 9). Silver likely plays a role in the C(sp)–H activation step since it could coordinate with the alkynyl group [46] , [47] , [48] . Solvent effects were also investigated in this transformation. Without additional solvent, the reaction yield decreased significantly ( Table 1 , entry 10). Benzene gave a similar result with chlorobenzene ( Table 1 , entry 11). Different oxidants were also applied in this transformation. Dicumyl peroxide could furnish the desired product in a lower yield ( Table 1 , entry 12). Benzoyl peroxide was not suitable in this transformation ( Table 1 , entry 13). In addition, the influence of temperature was also explored. Both decreased and increased temperatures gave decreased yields ( Table 1 , entries 14–15). It is worthy of note that oligomerization of 2a was the major side reaction pathway in all the above conditions. Table 1 Effects of reaction parameters. 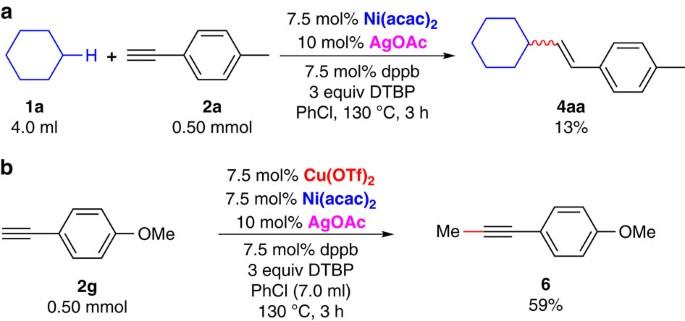Figure 2: Control experiments. (a) Addition to terminal alkyne in the absence of copper catalyst. (b) Direct methylation of terminal alkyne in the absence of alkane substrates. Full size table Figure 2: Control experiments. ( a ) Addition to terminal alkyne in the absence of copper catalyst. ( b ) Direct methylation of terminal alkyne in the absence of alkane substrates. Full size image Scope of unactivated alkanes To further demonstrate the applicability of this transformation, the reaction system was applied to other unactivated alkanes for the synthesis of substituted alkynes ( Fig. 3 ). Both cyclohexane and methylcyclohexane showed a good reaction efficiency toward alkynylation ( 3aa and 3ba ). Other cycloalkanes were applied as substrates in this transformation. The ring size had evident effect on the yield of the corresponding alkynylation products. For example, cyclopentane and cycloheptane did furnish the desired products but with decreased reaction efficiency ( 3ca and 3da ). Unactivated acyclic alkanes including linear alkanes and branched alkanes were tested in this oxidative C(sp 3 )–H alkynylation reaction. The reaction of 2a with linear alkanes including n -pentane, n -hexane and n -heptane proceeded smoothly but afforded a mixture of regioisomers ( 3ea – 3ga ). The reaction result of a branched alkane was also presented. Neohexane was also able to couple with 2a and afforded the desired product as two regioisomers ( 3ha ). Oxidative C(sp 3 )–H alkynylation of norbornane proceeded with single-site selectivity and gave 3ia in 49% yield. Despite simple alkanes, toluene derivatives were also suitable in this transformation. Direct oxidative benzylic C(sp 3 )–H alkynylation of toluene derivatives could be obtained in good yields under similar conditions ( 3ja–3la ). Since tert -butoxyl radical can undergo β–Me scission to generate a methyl radical [49] , [50] , [51] , [52] , direct methylation of terminal alkyne was observed as a competing side reaction in the above cases. Importantly, efficient methylation of terminal alkyne could be achieved in the absence of alkane substrates ( Fig. 2b ). 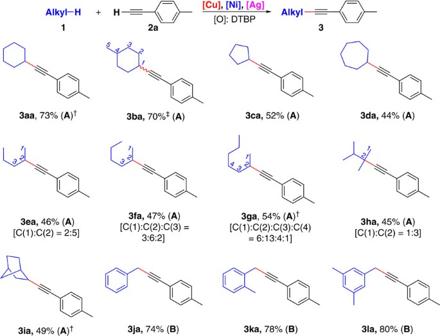Figure 3: Scope of alkanes substrates. Reaction conditionsA:1(4.0 ml),2a(0.50 mmol), Cu(OTf)2(7.5 mol%), Ni(acac)2(7.5 mol%), AgOAc (10 mol%), dppb (7.5 mol%) and DTBP (2.0 mmol), PhCl (3.0 ml), 130 °C, 3 h. The ratio of regioisomers shown in parentheses was determined by GC–MS. Reaction conditionsB:1(7.0 ml),2a(0.50 mmol), Cu(OTf)2(10 mol%), Ni(acac)2(10 mol%), AgOAc (5 mol%), dppb (10 mol%) and DTBP (0.75 mmol), 130 °C, 3 h.†DTBP (1.5 mmol) was used.‡Yields of all regioisomers. Figure 3: Scope of alkanes substrates. Reaction conditions A: 1 (4.0 ml), 2a (0.50 mmol), Cu(OTf) 2 (7.5 mol%), Ni(acac) 2 (7.5 mol%), AgOAc (10 mol%), dppb (7.5 mol%) and DTBP (2.0 mmol), PhCl (3.0 ml), 130 °C, 3 h. The ratio of regioisomers shown in parentheses was determined by GC–MS. Reaction conditions B: 1 (7.0 ml), 2a (0.50 mmol), Cu(OTf) 2 (10 mol%), Ni(acac) 2 (10 mol%), AgOAc (5 mol%), dppb (10 mol%) and DTBP (0.75 mmol), 130 °C, 3 h. † DTBP (1.5 mmol) was used. ‡ Yields of all regioisomers. Full size image Scope of terminal alkynes Different terminal alkynes were applied as substrates to react with cyclohexane ( Fig. 4 ). The reactions of simple phenylacetylene, meta - and ortho -methyl substituted phenylacetylene all proceeded well and afforded the corresponding aliphatic internal alkynes in good yields ( 3ab and 3ad ). 4–Ethynyl–1,1′–biphenyl also gave the desired products in good yields ( 3ae ). To our delight, electron-rich phenylacetylenes were more reactive, furnishing the desired products in higher yields ( 3af and 3ag ). At the same time, strongly electron-deficient phenylacetylenes were also suitable but with slightly decreased efficiency in this reaction system ( 3ah and 3ai ). It is noteworthy that silver had evident effect on the reaction yield of electron-deficient phenylacetylenes. For example, the yield of 3ah decreased markedly (14%) in the absence of AgOAc. Notably, halide substituents such as F, Cl and Br were all tolerated in this transformation, which provides the possibility for further functionalization ( 3aj – 3am ). Other aromatic alkynes were also applied in this transformation. 2-ethynylnaphthalene and 2-ethynylthiophene both furnished the desired products in good yields ( 3an and 3ao ). Delightfully, aliphatic alkyne such as 1-heptyne and cyclohexylacetylene were also suitable in the oxidative C(sp 3 )–H/C(sp) cross-coupling and afforded the desired product in good to excellent yields ( 3ap and 3aq ). Late-stage modification of a bioactive molecule is highly important for medical chemistry studies. Delightfully, 3-ethynylestrone containing carbonyl group and four continuous chiral centres furnished the desired coupling product in 70% yield under the standard conditions ( 3ar ). 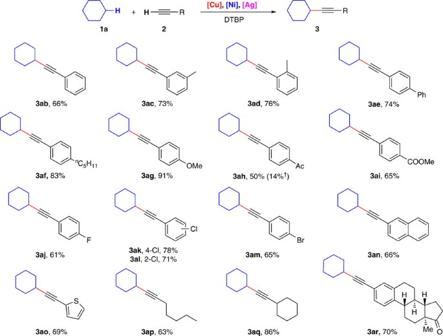Figure 4: Scope of terminal alkynes. Reaction conditions:1a(4.0 ml),2(0.50 mmol), Cu(OTf)2(7.5 mol%), Ni(acac)2(7.5 mol%), dppb (7.5 mol%), AgOAc (10 mol%) and DTBP (1.5 mmol), PhCl (3.0 ml), 130 °C, 3 h. Isolated yields are shown.†In the absence of AgOAc. Figure 4: Scope of terminal alkynes. Reaction conditions: 1a (4.0 ml), 2 (0.50 mmol), Cu(OTf) 2 (7.5 mol%), Ni(acac) 2 (7.5 mol%), dppb (7.5 mol%), AgOAc (10 mol%) and DTBP (1.5 mmol), PhCl (3.0 ml), 130 °C, 3 h. Isolated yields are shown. † In the absence of AgOAc. Full size image Since the method had been established, we then tried to gain some insights into the catalytic pathway. To confirm the existence of radical intermediates, a radical trapping experiment was carried out by using 1 equiv of (2, 2, 6, 6–tetramethylpiperidin–1–yl)oxy (TEMPO). No cross-coupling product 3aa was obtained in this reaction ( Fig. 5 ). Instead, the GC–MS and 1 H NMR analysis of the reaction mixture showed the existence of cyclohexyl radical trapped by TEMPO ( Supplementary Figs 66,67 ). 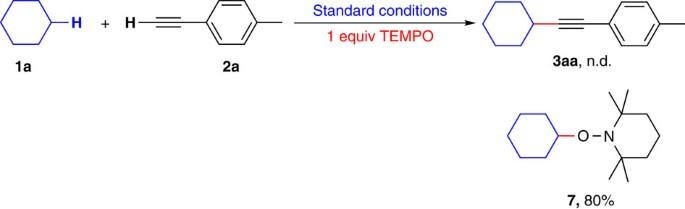Figure 5: Radical trapping experiment. Observation of trapped cyclohexyl radical. Figure 5: Radical trapping experiment. Observation of trapped cyclohexyl radical. Full size image Next, kinetic isotopic effect studies with separate kinetic experiments were performed to gain insights into the rate-determining step for this C–H/C–H cross-coupling reaction. Both the C(sp 3 )–H bond cleavage of 1a and the C(sp)–H bond cleavage of 2a were studied. A primary kinetic isotopic effect was observed for C(sp 3 )–H bond cleavage ( Fig. 6a , k H /k D =2.2) while no obvious kinetic isotopic effect was observed for the C(sp)–H cleavage ( Fig. 6b , k H /k D =0.9), suggesting that C(sp 3 )–H bond cleavage was probably the rate-determining step in this transformation (for details, see Supplementary Fig. 68 ) [53] . 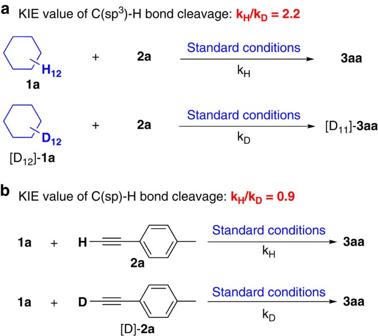Figure 6: Kinetic isotope effect experiments. (a) The initial reaction rate of1awith2a, [D12]–1awith2a. (b) The initial reaction rate of1awith2a,1awith [D]–2a. Figure 6: Kinetic isotope effect experiments. ( a ) The initial reaction rate of 1a with 2a , [D 12 ]– 1a with 2a . ( b ) The initial reaction rate of 1a with 2a , 1a with [D]– 2a . Full size image In the next step, the reactions with alkynyl metal species were performed to get some insights into the radical cross-coupling step. (Phenylethynyl)copper (2d–[Cu]) and (phenylethynyl)silver (2d–[Ag]) were prepared and used as substrates to react with 1a under the standard conditions ( Fig. 7 ). However, neither of them could furnish the cross-coupling product. Thus, both alkynyl Cu(I) complex and alkynyl Ag(I) complex are not likely to be involved in the C(sp 3 )–C(sp) cross-coupling process. An alkynyl Cu(II) complex is more possibly to be generated in this transformation. 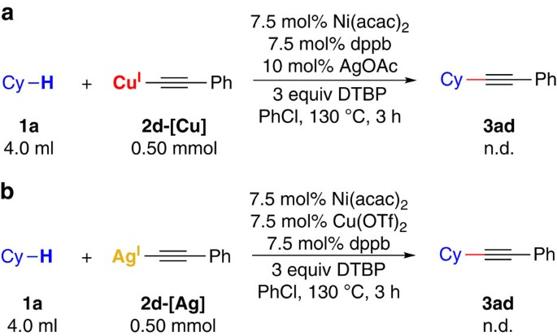Figure 7: Reactions of cyclohexane with alkynyl metal species. (a) Reaction between1aand2d–[Cu]under standard conditions. (b) Reaction between1aand2d–[Ag]under standard conditions. Figure 7: Reactions of cyclohexane with alkynyl metal species. ( a ) Reaction between 1a and 2d–[Cu] under standard conditions. ( b ) Reaction between 1a and 2d–[Ag] under standard conditions. Full size image On the basis of the experimental results and previous reports [50] , [51] , a plausible reaction mechanism is presented in Fig. 8 . Copper and silver work synergistically in the C(sp)–H activation of terminal alkyne, which leads to the formation of an alkynyl Cu(II) complex. The alkynyl copper complex is then transmetaled with Ni(II) species to generate an alkynyl Ni(II) complex. At the same time, an alkyl radical can be generated through hydrogen abstraction by in situ generated tert -butoxyl radical. This radical then reacts with the Ni(II) alkynyl complex [54] , [55] , [56] , [57] , [58] , [59] . The C(sp 3 )–C(sp) bond can be formed either through radical homolytic substitution or reductive elimination (see Supplementary Fig. 69 for details). Finally, the released Ni(I) species can be oxidized to Ni(II) species by DTBP to complete the nickel catalytic cycle. 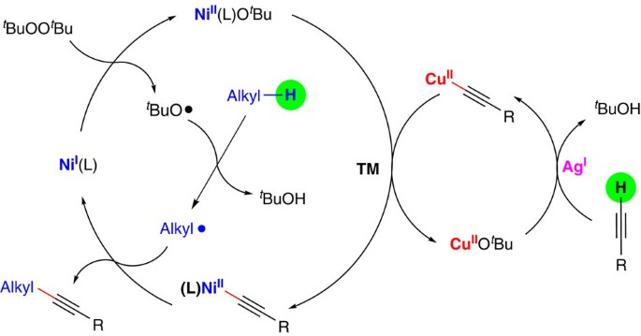Figure 8: Proposed catalytic cycles for the radical alkynylation reaction through multimetallic catalysis. Tentative reaction mechanism involves oxidation of alkane to generate an alkyl radical, silver-assisted copper(II)-acetylide formation, transmetalation with nickel, and finally C(sp3)–C(sp) bond formation. Figure 8: Proposed catalytic cycles for the radical alkynylation reaction through multimetallic catalysis. Tentative reaction mechanism involves oxidation of alkane to generate an alkyl radical, silver-assisted copper(II)-acetylide formation, transmetalation with nickel, and finally C(sp 3 )–C(sp) bond formation. Full size image In conclusion, we have developed a combined Cu/Ni/Ag catalytic system to achieve the challenging oxidative C(sp 3 )–H/C(sp)–H cross-coupling of unactivated alkanes with terminal alkynes. The utilization of multimetallic catalysis was the key for controlling the reaction selectivity toward C(sp 3 )–C(sp) bond formation. Various substituted alkynes were synthesized in good to high yields with a good functional group tolerance. Preliminary mechanistic studies suggest that the reaction proceeds through a transition-metal-catalysed radical reaction pathway and that the C(sp 3 )–H bond cleavage of unactivated alkanes is the rate-limiting step. This work not only provides an environmentally friendly approach to access alkyne compounds, but also contributes new knowledge to radical cross-coupling chemistry. The application of the radical alkynylation strategy in the synthesis of other substituted alkynes is underway in our laboratory. General procedure (3aa) In an oven-dried Teflon septum screw-capped tube equipped with a stir bar, Cu(OTf) 2 (13.6 mg, 0.038 mmol), Ni(acac) 2 (9.6 mg, 0.038 mmol), dppb (16.0 mg, 0.038 mmol) and AgOAc (8.3 mg, 0.050 mmol) were combined and sealed. The tube was then charged with nitrogen. Then cyclohexane (4.0 ml) and PhCl (3.0 ml) were injected into the tube by syringe. After stirring for 5 min, DTBP (135 mg, 1.5 mmol) and p -tolylacetylene (58.0 mg, 0.50 mmol) were subsequently injected into the reaction tube. The reaction was then heated to 130 °C. After stirring for 3 h, the reaction was cooled down to room temperature and quenched with saturated Na 2 S 2 O 3 solution. After extraction with ethyl acetate (3 × 10 ml), the organic layers were combined and dried over anhydrous Na 2 SO 4 , the pure product was obtained by flash column chromatography on silica gel (petroleum:ethyl ether=10:1). Colourless oil was obtained in 73% isolated yield. 1 H NMR (400 MHz, CDCl 3 ) δ 7.28 (d, J =8.1 Hz, 2H), 7.06 (d, J =7.9 Hz, 2H), 2.56 (tt, J =9.0, 3.6 Hz, 1H), 2.31 (s, 3H), 1.92–1.82 (m, 2H), 1.80–1.69 (m, 2H), 1.59–1.46 (m, 3H), 1.40–1.28 (m, 3H). 13 C NMR (101 MHz, CDCl 3 ) δ 137.26, 131.38, 128.84, 120.99, 93.58, 80.47, 32.75, 29.65, 25.92, 24.90, 21.34. For 1 H NMR, 13 C NMR, 19 F NMR and GC–MS (if applicable) spectra of compounds 3aa-3la , 3ab–3ar , 6 see Supplementary Figs 1–66 . For the general information of the analytical methods and the mechanistic studies, please see Supplementary Methods . Data availability The authors declare that the data supporting the findings of this study are available within the article and its Supplementary Information files. How to cite this article: Tang, S. et al . Multimetallic catalysed radical oxidative C(sp 3 )–H/C(sp)–H cross-coupling between unactivated alkanes and terminal alkynes. Nat. Commun. 7:11676 doi: 10.1038/ncomms11676 (2016).